Replication of flexible polymer membranes with geometry-controllable nano-apertures via a hierarchical mould-based dewetting Membranes with nano-apertures are versatile templates that possess a wide range of electronic, optical and biomedical applications. However, such membranes have been limited to silicon-based inorganic materials to utilize standard semiconductor processes. Here we report a new type of flexible and free-standing polymeric membrane with nano-apertures by exploiting high-wettability difference and geometrical reinforcement via multiscale, multilevel architecture. In the method, polymeric membranes with various pore sizes (50–800 nm) and shapes (dots, lines) are fabricated by a hierarchical mould-based dewetting of ultraviolet-curable resins. In particular, the nano-pores are monolithically integrated on a two-level hierarchical supporting layer, allowing for the rapid (<5 min) and robust formation of multiscale and multilevel nano-apertures over large areas (2 × 2 cm 2 ). Free-standing nano-membranes have been fabricated from various materials, such as Si-based inorganics [1] , [2] , [3] , [4] , [5] , [6] , thin metal foils [7] , [8] and other types of nano-materials [9] , [10] , [11] , [12] , [13] , [14] , for use in a wide range of applications including shadow masking [3] , [4] , molecular separation [5] , [6] , [15] , plasmonics [4] , [7] , energy devices [16] , [17] , [18] and bio-inspired microfluidic devices [19] , [20] . In general, a series of standard semiconductor processes and/or specific materials [7] , [21] with high mechanical rigidity have been required to maintain the membrane’s shape firmly without mechanical fracture or tear against external forces that arise during the handling process. For example, a highly robust SiN x (Young’s modulus, E >130 GPa) nano-membrane was formed on top of a rigid silicon support via electron-beam lithography or focused ion-beam milling [3] , [4] , [6] . Such a thin SiN x membrane is known to be complicated and expensive to fabricate, and fragile under mechanical contact or moisture at ambient conditions. In parallel, a template-based bottom-up method is useful to create a free-standing membrane with nano-apertures integrated on a geometrical support by utilizing self-assembly of nano-particles [22] or block copolymers [23] . The ability to control the aperture shape or dimension, however, is potentially limited, restricting the widespread use of such a template-mediated approach. In addition, an interesting method for generation of complex hierarchical pillars with high aspect ratio was reported, but the robust fabrication of free-standing and flexible membranes having ordered hierarchical apertures still remains challenging [24] . Alternatively, elastomeric polydimethylsiloxane membranes with microscale pores (>5 μm) have been used by spin-coating and replica moulding from micropillar arrays [19] , [25] , [26] , [27] , [28] . As the polydimethylsiloxane membranes offer several advantages such as conformal wetting and easy peel-off without significant damage and distortion, they have been employed as a shadow mask for the patterning of a variety of materials: from electroluminescent materials [25] to carbon-based nano-materials such as graphene, carbon nano-tubes and fullerenes [28] . Nonetheless, polymeric membranes with nano-apertures have rarely been reported owing in part to the fact that they are required to be ‘free standing’ and ‘residual-layer-free’, which are difficult to achieve with the existing polymers and fabrication processes. In particular, the low elastic modulus of soft polymers causes tears and defects in the membrane during the fabrication or handling process. It is also not easy to remove the residual layer to produce clear through-holes; thus, additional etching or specific skills have been required [29] , [30] , [31] , [32] , [33] . To address these challenges, we present a simple, yet robust replication method to create a new type of flexible and free-standing polymeric membrane with geometry-controllable nano-pores by a hierarchical mould-based dewetting. Our material-based strategy combines large affinity (or wettability) difference in micromoulding and geometric reinforcement via multiscale, multilevel architecture. Especially, the method involves spontaneous dewetting of a hydrophobic (hydrophilic), ultraviolet (UV)-curable resin against a hydrophilic (hydrophobic) mould, which is significantly amplified by the hierarchical geometry of the mould. Moreover, a simple theory is developed to ensure mechanical stability of nano-apertures in bridge shapes without structural collapses, which could be used as a guide for the design of robust polymeric nano-aperture engineering. Binary dewetting process by using a hierarchical mould A schematic illustration for the fabrication of a polymer membrane with two-level apertures is shown in Fig. 1a , in which representative scanning electron microscopy (SEM) images of the bottom dual-scale mould (150-nm pillars on 20-μm microposts) are shown in the lower panel. The key idea is to utilize a hierarchical mould-based dewetting process in a sandwich assembly consisting of upper and lower moulds; first, a UV-curable hydrophobic polymer resin (for example, perfluoropolyether (PFPE)) is confined between a lower two-level hierarchical mould and a flat upper blanket made of a hydrophilic polymer resin (for example, polyurethane acrylate (PUA)), and subsequently cured and separated in a short period of time (<2 min), leaving behind the exposed top surface of PUA nano-pillars without a residual layer of PFPE. It is noted in this regard that a typical nano-imprinting or moulding process gives rise to a thick residual layer even with materials with a large affinity difference, which needs to be removed by a subsequent dry or wet etching process. Supplementary Fig. 1a,b shows a residual layer made in a typical moulding process even under a physical load of ~20 N cm −2 . Supplementary Fig. 1c also shows a nano-membrane with an array of 450-nm pores leaving behind many cracks and defects made during a simple moulding process without using the present concept of the hierarchical mould-based dewetting process. Although a replication process was performed using a natural hierarchical template that diatom biosilica has, there remained a residual layer under the replicated patterns [34] . The more important and unique feature of our method is the capability of generating non-residual layer and free-standing membranes by exploiting not only a high-wettability difference but also a utilization of a hierarchical structure as a mould. Here, the two-level hierarchical mould can be made by a two-step moulding process utilizing oxygen inhibition effects [35] , [36] or conventional multilevel photolithography [37] . 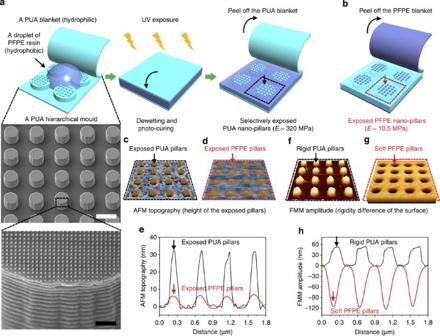Figure 1: The dewetting-induced micromoulding process. (a,b) Micromoulding of a hydrophobic PFPE resin within a sandwich assembly between a two-level hydrophilic PUA mould and a flat PUA blanket (a). The materials can be swapped with the same procedure to obtain a dewetting surface of PUA (b). Representative SEM images of the two-level bottom mould (150 nm/20 μm) are shown in the lower panel. Scale bar, 30 μm (white), 1 μm (black). (c–h) Analysis of the spatial distribution of topography (c–e) and rigidity (f–h) of the dewetted surface with two exposed PUA (c,f, black line ine,h) and PFPE (d,g, red line ine,h) pillars. The FMM data clearly show complete exposure of the PUA pillars with the background of the PFPE (f), and vice versa (g). Figure 1: The dewetting-induced micromoulding process. ( a , b ) Micromoulding of a hydrophobic PFPE resin within a sandwich assembly between a two-level hydrophilic PUA mould and a flat PUA blanket ( a ). The materials can be swapped with the same procedure to obtain a dewetting surface of PUA ( b ). Representative SEM images of the two-level bottom mould (150 nm/20 μm) are shown in the lower panel. Scale bar, 30 μm (white), 1 μm (black). ( c – h ) Analysis of the spatial distribution of topography ( c – e ) and rigidity ( f – h ) of the dewetted surface with two exposed PUA ( c , f , black line in e , h ) and PFPE ( d , g , red line in e , h ) pillars. The FMM data clearly show complete exposure of the PUA pillars with the background of the PFPE ( f ), and vice versa ( g ). Full size image When a UV-curable resin is drop-dispensed on a two-level hierarchical mould with a blank layer of the same material, the resin spontaneously spreads inside the confined spaces and a majority of the resin is squeezed out of the assembly on an applied pressure with the aid of the large affinity difference (‘dewetting’). It is interesting to note that dewetting is not dependent on the amount of drop-dispensed resin, because the employment of both hydrophobic (or hydrophilic) hierarchical moulds in the sandwich-like moulding process for hydrophilic (or hydrophobic) resin induces a conformal contact by quickly expelling the excessive resins from the set-up. This means that there is no residual layer and therefore, the membrane thickness is not dependent on the amount of drop-dispensed resins after a peel-off process. After separation of the blank layer, the exposed PUA pillars are clearly observed with the background of the PFPE polymer. In our experiment, the hydrophilic PUA [34] , [35] was mostly used as upper and lower moulds in order to replicate the hydrophobic PFPE resins [38] , [39] , [40] ; the materials can be swapped to obtain the exposed PFPE pillars with the background of the dewetted PUA domain ( Fig. 1b ). Although not shown, the PFPE mould could even dewet a highly viscous (140 cps) Norland Optical Adhesive (NOA73) [41] and other UV-curable resins in the same one-step moulding process. Characterization of the dewetting surfaces To verify the direct exposure of the dewetting interface, detailed binary mechanical mappings were performed using atomic force microscopy (AFM) and force modulation microscopy (FMM). In this way, one can probe the rigidity distribution between the exposed nano-pillars and the dewetting surface ( Fig. 1c–h ). According to the AFM topographic images ( Fig. 1c–e ), the exposed heights of the PFPE and PUA nano-pillars after dewetting were ~7 nm and ~32 nm, respectively. Such a difference of the exposed heights may be attributed to different shrinkage of the two resins in the curing, in addition to a local affinity difference at the three-phase interface. In order to investigate the exact material distribution, detailed binary mappings were carried out using FMM, since the exposed PUA or PFPE pillars have different mechanical properties (for example, Young’s modulus of PUA: 320 MPa, PFPE: 10.5 MPa). It is known that when the tip contacts a hard surface, a large amplitude response occurs by an amplification of the oscillation. On the other hand, a small amplitude response is expected on a soft surface by an absorbance of the oscillation. As shown in Fig. 1f–h , the amplitudes on the dewetting surface were ~+50 nm for the rigid PUA and ~−110 nm for the soft PFPE, respectively, suggesting that the two materials are indeed separated in two distinct domains via spontaneous dewetting. Two-level apertures in a free-standing polymeric membrane A notable advantage in the current approach is the generation of robust polymeric multilevel nano-apertures by directly integrating a seemingly fragile membrane into a microscale backbone. To demonstrate the geometrical reinforcement, we directly peeled off the dewetting membrane from the assembly, yielding a PFPE membrane having high-density 450-nm clear through-holes supported on a membrane with 60-μm rectangular patterns as shown in Fig. 2a . The SEM images in Fig. 2b suggest that the membrane is sufficiently robust and stable owing to the geometrical reinforcement by leveling, which is similar to various thin nano-material membranes supported on geometrical backbones reported earlier by many researchers [11] , [12] , [42] . 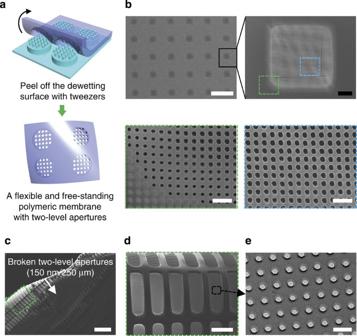Figure 2: Direct replication of two-level apertures. (a) Illustration of the peel-off process from the dewetting surface to obtain a flexible and free-standing membrane with two-level apertures. (b) SEM images of the 450-nm apertures on a microscale backbone of 60-μm holes at different magnifications. Scale bar, 200 μm (white) and 10 μm (black). The magnified images show clear through-holes of the membrane in the boxed regions (blue and green). Scale bar, 2 μm. (c) SEM image showing the broken areas with 150-nm apertures with a magnified view of the boxed region (green) (d). Scale bar in (c) and (d) are 600 μm and 100 μm, respectively. (e) Transmission electron microscopy image of the boxed region, showing an array of clear through-holes of 150-nm diameter. Scale bar, 600 nm. Figure 2: Direct replication of two-level apertures. ( a ) Illustration of the peel-off process from the dewetting surface to obtain a flexible and free-standing membrane with two-level apertures. ( b ) SEM images of the 450-nm apertures on a microscale backbone of 60-μm holes at different magnifications. Scale bar, 200 μm (white) and 10 μm (black). The magnified images show clear through-holes of the membrane in the boxed regions (blue and green). Scale bar, 2 μm. ( c ) SEM image showing the broken areas with 150-nm apertures with a magnified view of the boxed region (green) ( d ). Scale bar in ( c ) and ( d ) are 600 μm and 100 μm, respectively. ( e ) Transmission electron microscopy image of the boxed region, showing an array of clear through-holes of 150-nm diameter. Scale bar, 600 nm. Full size image There is a potential limitation with the two-level architecture in replicating a high-density array of nano-apertures (~150 nm in diameter) over a large area. When the base size of the microscale backbone was increased to rectangular holes of 60 × 250 μm 2 , many broken regions were seen as shown in Fig. 2c , which is associated with a reduced thickness of nano-apertures. As described in Fig. 1e , the exposed height of the PUA nano-pillar (the height of nano-pillar is about 200 nm) was ~32 nm, indicating that the thickness of PFPE nano-apertures is merely ~168 nm, which is deemed low to ensure good mechanical stability of 150-nm pores over the patterned field of 60 × 250 μm 2 . As a result, many defects like cracks and tears were mostly observed at the boundary of nano-apertures after the ‘peel-off’ process. Nonetheless, the SEM image and the transmission electron microscopy image in Fig. 2d,e show an array of clear through-holes of 150-nm diameter in the centre location. This finding leads us to propose a design principle such that a three-level architecture would be more appropriate to make a robust polymeric membrane with sub-100-nm nano-apertures, which is described below. Polymeric membrane with three-level nano-apertures In order to create a membrane with three-level nano-apertures, a nano-patterned upper mould with various pattern sizes and shapes (dots or lines) was used instead of a flat blanket as illustrated in Fig. 3a . After the same back-filling, curing and disintegration of the assembly, a three-level nano-membrane could be neatly formed in the one-step moulding process within 5 min. 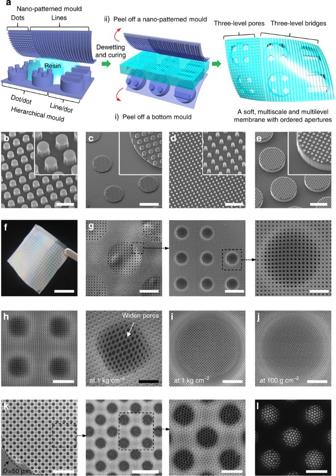Figure 3: Fabrication of a robust membrane with three-level apertures. (a) Illustration for the fabrication of a membrane with geometry-tunable three-level nano-apertures. Various nano-apertures in the form of pores or lines can be incorporated into the polymeric membrane. (b–e) SEM images of single-scale (bandd, 800-nm pillars and 150-nm pillars, respectively; scale bar, 2 μm) and dual-scale hierarchical moulds (cande, 20 μm/500 μm and 5 μm/150 μm posts; scale bar, 500 μm and 100 μm, respectively). (f–k) Large-area digital (f) and SEM images (g–k) of the three-level apertures demonstrating that the nano-pores are well defined without structural collapses or defects: 800-nm/20-μm/500-μm apertures (g) and 150-nm/5-μm/150-μm apertures (h) at different magnifications. Scale bar, 1 cm in (f). Scale bar in (g) are 250 μm, 25 μm and 5 μm from left to right, respectively. Scale bar, 5 μm (white) and 2 μm (black) in (h). Owing to the stress concentration, some widened apertures (>150 nm) were observed under an applied pressure of 1 kg cm−2. (i,j) Aperture size modulation by controlling the stress concentration where a different two-level hierarchal mould (20 μm/500 μm) was used under the same pressure (i) and a reduced pressure of 100 g cm−2was used (j). Scale bar, 5 μm. (k) SEM images of 50-nm/800-nm/50-μm apertures at different magnifications. Scale bar in (k) are 5 μm, 2 μm and 800 nm from left to right, respectively. (l) SEM image of multiscale Au dot patterns using the aperture as a shadow mask. Scale bar, 800 nm. Figure 3b–e shows SEM images of single-scale (b,d) and dual-scale hierarchical moulds (c,e) used to create three-level apertures, with the diameter of nano-pores ranging from 800 to 50 nm. For example, 800-nm posts ( Fig. 3b ) and 20-μm posts/500-μm posts ( Fig. 3c ) were combined to fabricate the three-level apertures of 800 nm/20 μm/500 μm (from top to bottom). Similarly, 150-nm posts ( Fig. 3d ) and 5-μm posts/150-μm posts ( Fig. 3e ) were chosen for the three-level apertures of 150 nm/5 μm/150 μm. For easy handling of extremely tiny apertures, the lower two-level aperture plays an important role as the geometrical reinforcement, which enables large-area (~2 × 2 cm 2 ) fabrication with high mechanical stability ( Fig. 3f ). Figure 3g shows an example of three-level pores (diameter: 800 nm/20 μm/500 μm) at different magnifications where the dimples were formed on the entire surface in the moulding process, while clear through-holes were seen within the 20-μm second-level pores. Figure 3: Fabrication of a robust membrane with three-level apertures. ( a ) Illustration for the fabrication of a membrane with geometry-tunable three-level nano-apertures. Various nano-apertures in the form of pores or lines can be incorporated into the polymeric membrane. ( b – e ) SEM images of single-scale ( b and d , 800-nm pillars and 150-nm pillars, respectively; scale bar, 2 μm) and dual-scale hierarchical moulds ( c and e , 20 μm/500 μm and 5 μm/150 μm posts; scale bar, 500 μm and 100 μm, respectively). ( f – k ) Large-area digital ( f ) and SEM images ( g – k ) of the three-level apertures demonstrating that the nano-pores are well defined without structural collapses or defects: 800-nm/20-μm/500-μm apertures ( g ) and 150-nm/5-μm/150-μm apertures ( h ) at different magnifications. Scale bar, 1 cm in ( f ). Scale bar in ( g ) are 250 μm, 25 μm and 5 μm from left to right, respectively. Scale bar, 5 μm (white) and 2 μm (black) in ( h ). Owing to the stress concentration, some widened apertures (>150 nm) were observed under an applied pressure of 1 kg cm −2 . ( i , j ) Aperture size modulation by controlling the stress concentration where a different two-level hierarchal mould (20 μm/500 μm) was used under the same pressure ( i ) and a reduced pressure of 100 g cm −2 was used ( j ). Scale bar, 5 μm. ( k ) SEM images of 50-nm/800-nm/50-μm apertures at different magnifications. Scale bar in ( k ) are 5 μm, 2 μm and 800 nm from left to right, respectively. ( l ) SEM image of multiscale Au dot patterns using the aperture as a shadow mask. Scale bar, 800 nm. Full size image In the current approach, one can modulate the size of nano-pores by applying a different preload onto the assembly. For example, in the presence of an applied pressure, a large stress would be delivered to the region containing nano-pores while the pillars are further squeezed, resulting in the formation of wider apertures than the original ones. This is well represented in Fig. 3h , where the widened apertures (>200 nm) are formed on a two-level support of 5 μm/150 μm pores under the pressure of ~1 kg cm −2 . One can alleviate this problem with two approaches by selecting a hierarchical mould with a larger micro-patterned region in order to distribute the stress uniformly or minimizing the applied pressure to reduce the stress concentration. For the former, a hierarchical mould of 20 μm/500 μm was used instead under the same pressure condition (1 kg cm −2 ), yielding highly uniform arrays of 180-nm apertures ( Fig. 3i ). For the latter, a smaller pressure (~100 g cm −2 ) was applied to the assembly and exact 150-nm pores with the same size of dimples were observed with good uniformity ( Fig. 3j ). To further reduce the pore size below 100 nm, a PFPE mould with nano-pillars of ~50 nm diameter was replicated from the surface-treated anodic aluminium oxide template [43] . Following the same procedure with the PUA resin along with the PFPE upper and lower moulds, a membrane with three-level pores (50 nm/800 nm/50 μm) was obtained ( Fig. 3k ). It should be noted that a two-level architecture may not be suitable to replicate these tiny nano-pores as mentioned earlier (see Fig. 2c ). According to the three-level hierarchical geometry, the density of 50-nm pores was ~1.17 × 10 9 cm −2 , which seems challenging with the electron-beam lithography or focused ion-beam process currently used for fabricating nano-apertures on a silicon-based inorganic membrane. Also, this polymeric membrane has the potential for its use as a shadow mask, as clearly demonstrated in the formation of dual-scale Au arrays on a silicon substrate shown in Fig. 3l . Membrane with asymmetric pores and stability criterion To elaborate on the mechanical stability of nano-apertures, various nano-patterned moulds having pillars and/or lines were prepared using the same procedure. First, a PFPE mould with parallel 70-nm lines was placed onto a PFPE hierarchical mould having two-level dots (800 nm/50 μm). This allows for the replication of a membrane of the three-level pores made of the PUA resin as shown in Fig. 4a at different magnifications. If we select larger second-level pores of 5 μm diameter to make longer parallel bridges, some lateral collapses will be observed in the form of mating between the neighbouring bridges ( Fig. 4b ). 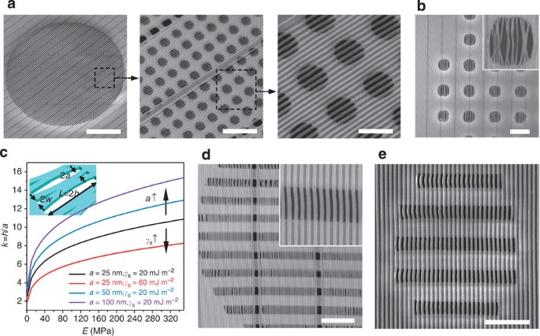Figure 4: Fabrication of various asymmetric nano-apertures and stability criterion. (a,b) Parallel nano-bridges on holey geometric backbones: 70-nm lines/800-nm pores/50-μm pores (a) and 70-nm lines/5-μm pores/150-μm pores (b). Scale bar in (a) are 15 μm, 3 μm and 500 nm from left to right, respectively. Scale bar, 15 μm in (b). Some lateral collapses are seen from the second-level pores of 5 μm in (b). (c) Plot ofk(=h/a) as a function ofE. Similarly, asymmetric rectangular pores can be made by rotating the upper mould by 90° with respect to the lower mould: 70-nm lines/800-nm lines/50-μm pores (d) and 550-nm lines/3-μm lines/50-μm pores (e). Scale bar in (d) and (e) are 3 μm and 10 μm, respectively. In order to explain this observation, the stability criterion can be derived for the parallel line arrays, which is given by [44] Figure 4: Fabrication of various asymmetric nano-apertures and stability criterion. ( a , b ) Parallel nano-bridges on holey geometric backbones: 70-nm lines/800-nm pores/50-μm pores ( a ) and 70-nm lines/5-μm pores/150-μm pores ( b ). Scale bar in ( a ) are 15 μm, 3 μm and 500 nm from left to right, respectively. Scale bar, 15 μm in ( b ). Some lateral collapses are seen from the second-level pores of 5 μm in ( b ). ( c ) Plot of k (= h / a ) as a function of E . Similarly, asymmetric rectangular pores can be made by rotating the upper mould by 90° with respect to the lower mould: 70-nm lines/800-nm lines/50-μm pores ( d ) and 550-nm lines/3-μm lines/50-μm pores ( e ). Scale bar in ( d ) and ( e ) are 3 μm and 10 μm, respectively. Full size image where 2 a is the line width, 2 w is the space between lines, 2 h (= L ) is the length of parallel bridges, E * is the effective Young’s modulus, being approximated to 4 E /3 and γ s is the surface energy of polymer. For simplicity, a dimensionless parameter can be defined, k ≡ h/a = L /2 a , which allows us to estimate the maximum length of nano-bridges without structural collapses ( L=k × 2 a ). For the equal line-and-space pattern ( a=w ), it follows that We tested four kinds of UV-curable polymers with various ranges of surface energy (20–60 mJ m −2 ) and elastic modulus (10–320 MPa) (see Table 1 ). According to the above criterion ( Fig. 4c ), in the case of nano-bridges with the soft PUA301 material, the range of k is 5–6 when the width of nano-lines ranges from 50 to 100 nm; this means self-mating would occur at L ~385 nm for 70-nm lines ( k ~5.5). If we choose the hard PUA311, the value of k is much elevated to 10–12 under the same conditions (2 a =50–100 nm) despite that these two materials have similar surface properties. In this case, the mating would occur at L ~770 nm assuming an average k value of 11. It is noted that no stability problem was observed for the circular pores regardless of the feature size. Table 1 Mechanical and surface properties of four ultraviolet-curable resins. Full size table On the basis of the above criterion, asymmetric apertures of rectangular shape were created by integrating two nano-bridges with the third-level aperture being rotated 90° with respect to the underlying two-level aperture. In detail, the 70-nm-width bridges were orthogonally aligned on arrays of parallel 800-nm bridges supported on 50-μm pore arrays as a backbone (three-level apertures, PUA311). Since we selected 800-nm lines (>770 nm) as the supporting backbone for the 70-nm bridges, some lateral collapses were observed between the neighbouring bridges ( Fig. 4d ). In contrast, the structures were stable and hardly interconnected for the 550-nm nano-bridges when supported on a 3-μm-line backbone ( Fig. 4e ). These design rules may be used as a guide to fabricate robust asymmetric rectangular-shaped pores or bridges on a free-standing and flexible membrane, which is potentially useful for tailoring the geometry of nano-apertures. Demonstration of serial shadow masking with an alignment As a potential application of the polymeric membrane with multilevel apertures, a step-and-repeat process was tested with a suitable alignment, where a PUA membrane with two-level parallel bridges of ~550 nm width was used. As shown in Fig. 5 , the membrane could be used twice to form multiscale Au patterns in a serial fashion under an alignment process ( Fig. 5a ). Remarkably, the nano-membrane was mechanically robust and self-wettable without tears or cracks after multiple peeling-offs in the attaching and detaching processes more than 20 times (see Supplementary Movie 1 ), offering direct evidence to the geometrical reinforcement of the multilevel architecture. Moreover, the attached membrane was fixed firmly and stably even with external disturbances, further supporting the robustness of the nano-membrane in multiple operations ( Fig. 5b–f ). 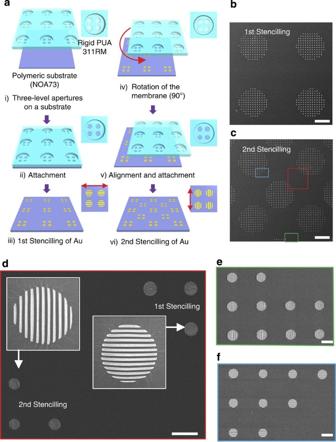Figure 5: Step-and-repeat process using polymeric membrane as a shadow mask. (a) Schematic illustration of the step-and-repeat stencilling of Au patterns (40 nm thickness) via a polymeric membrane with three-level parallel bridges (550-nm lines/10-μm pores/500-μm pores) onto a flexible polymer substrate (NOA73). (b–f) SEM images of the stenciling results after the 1st (b) and 2nd (c–f) deposition of Au layer. After the 1st stencilling, parallel nano-lines (550 nm) are generated on the substrate as shown in (b). Scale bar in (b) and (c) are 250 μm. By rotating the membrane by 90 degrees with an alignment process, arrays of multiscale perpendicular lines (550 nm) are also formed on the same substrate. Here, (d) is a magnified image of the red box in (c), (e,f) corresponds to the blue and green boxes in (c), respectively. Scale bar, 30 μm in (d) and 10 μm in (e) and (f). Figure 5: Step-and-repeat process using polymeric membrane as a shadow mask. ( a ) Schematic illustration of the step-and-repeat stencilling of Au patterns (40 nm thickness) via a polymeric membrane with three-level parallel bridges (550-nm lines/10-μm pores/500-μm pores) onto a flexible polymer substrate (NOA73). ( b – f ) SEM images of the stenciling results after the 1st ( b ) and 2nd ( c – f ) deposition of Au layer. After the 1st stencilling, parallel nano-lines (550 nm) are generated on the substrate as shown in ( b ). Scale bar in ( b ) and ( c ) are 250 μm. By rotating the membrane by 90 degrees with an alignment process, arrays of multiscale perpendicular lines (550 nm) are also formed on the same substrate. Here, ( d ) is a magnified image of the red box in ( c ), ( e , f ) corresponds to the blue and green boxes in ( c ), respectively. Scale bar, 30 μm in ( d ) and 10 μm in ( e ) and ( f ). Full size image Demonstration of emulsion reorganization via nano-apertures Owing to the facile handling of the soft membrane, our hierarchical membrane with nano-apertures was easy to be attached onto a tip of a syringe and strong enough (owing to hierarchical structure) to inject a liquid flow through each nano-aperture to reorganize nano-emulsions. Although a robust SiN membrane with nano-apertures may give simple pattering of metal atoms via apertures, a direct filtration or manipulation of liquid flow would be quite challenging owing to the cracking. 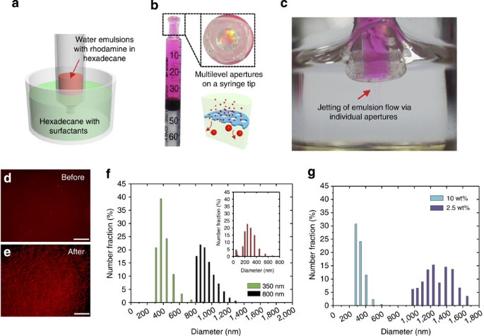Figure 6: Emulsion reorganizations via individual apertures in a polymeric membrane. (a) Schematic illustration of the reorganization steps via individual apertures. (b) Digital images of the integrated polymeric membrane onto a tip of a syringe, which indicates the facile utilization of the membrane in that the materials is sufficiently flexible to be embedded with any arbitrary surface. The inset illustration depicts the reorganization process near the apertures. (c) Digital image shows the streamline of jetting of emulsions during the reorganization process. A three-level membrane with hierarchical apertures (800 nm/20 μm/500 μm) was utilized to form a highly uniform emulsion. (d,e) Microscopic images with fluorescence probe (Rhodamine B) to show the size change of water emulsions before (d) and after (e) filtrations. Scale bar, 50 μm in (d) and (e). Note that the size of pre-emulsion is smaller than 300 nm, thus the individual emulsion could not be detected in the image. (f) Size distributions of emulsions before and after the filtration of apertures having two different diameter; 800-nm apertures and 350-nm apertures. (g) Dependence of emulsion size versus surfactant concentration for the case of a 800-nm pore membrane. Figure 6a shows a schematic illustration and experimental results of the reorganization process via an array of soft nano-apertures. As the membrane is based on the polymer (NOA73), it is quiet flexible to be attached and deformed around the tip ( Fig. 6b ). A sealing with commercial epoxy was done near the sidewall to prevent a leakage between the syringe and the membrane. After a preparation of a sample with pre-emulsions by the reported procedure [45] , we obtained a sample with polydispersive water emulsions (mean diameter: 261.9 nm) by mixing a small amount of water in hexadecane with an aid of surfactant (1:1 ratio of Span-20 and Tween-80). A liquid flow (1 ml min −1 ) through an array of multilevel apertures (800 nm/20 μm/500 μm) can provide jetting of emulsion flow via an individual aperture ( Fig. 6c , Supplementary Movie 2 ) and it should be noted that each micro jet flow through each nano-aperture can provide the same condition of shear-induced agglomeration for all apertures, which could yield uniform reorganization of emulsions. These results could be noticed by comparing the size of emulsions from the two microscopic images in Fig. 6d,e . To investigate the tendency of size changes, we performed a dynamic light scattering analysis with the emulsion sample ( Fig. 6f ). Here, highly uniform and skewed distributions of emulsions were obtained with a mean size depending on the pore size; for example, 800 nm pore and 350 nm pore generate the mean sizes 927.1 nm and 414.4 nm, respectively, when the concentration of surfactant in both a syringe and a beaker was same (5%). The dependency of pore size on the emulsion mean size is attributed to the mechanism based on shear-induced agglomeration [46] , which is proportional to shear rate and agglomeration time. While smaller diameter hole allows a nano-jet flow having a higher shear rate proportional inversely to the diameter, the agglomeration time that is directly proportional to the potential core length of the nano-jet flow should depend on the square of the pore diameter for a given velocity [47] . Therefore, agglomeration, which is proportional to shear rate times agglomeration time, would be linearly proportional to the diameter of pore. This means that a micro jet flow through a smaller sized pore experiences smaller agglomeration to yield smaller mean sizes of emulsions as shown in Fig. 6f . It is obvious that different concentrations of surfactants in the beaker strongly influence the agglomeration process. A smaller concentration (2.5 wt%) of surfactant compared with that (5 wt%) in the syringe resulted in the increase of emulsion sizes while a higher concentration (10 wt%) reduced the emulsion size ( Fig. 6g ). The demonstrated application takes advantage of our membrane containing many uniform size nano-apertures that can reorganize and generate highly uniform emulsions compared with the conventional method of nano-emulsion generation relying on self-assembly [48] , [49] . Figure 6: Emulsion reorganizations via individual apertures in a polymeric membrane. ( a ) Schematic illustration of the reorganization steps via individual apertures. ( b ) Digital images of the integrated polymeric membrane onto a tip of a syringe, which indicates the facile utilization of the membrane in that the materials is sufficiently flexible to be embedded with any arbitrary surface. The inset illustration depicts the reorganization process near the apertures. ( c ) Digital image shows the streamline of jetting of emulsions during the reorganization process. A three-level membrane with hierarchical apertures (800 nm/20 μm/500 μm) was utilized to form a highly uniform emulsion. ( d , e ) Microscopic images with fluorescence probe (Rhodamine B) to show the size change of water emulsions before ( d ) and after ( e ) filtrations. Scale bar, 50 μm in ( d ) and ( e ). Note that the size of pre-emulsion is smaller than 300 nm, thus the individual emulsion could not be detected in the image. ( f ) Size distributions of emulsions before and after the filtration of apertures having two different diameter; 800-nm apertures and 350-nm apertures. ( g ) Dependence of emulsion size versus surfactant concentration for the case of a 800-nm pore membrane. Full size image We have presented a robust fabrication method and design rules for a flexible, free-standing polymeric nano-membrane made of UV-curable polymers. The method involves a series of well-established steps via replica moulding, dewetting and UV photocrosslinking. It provides a simple, economically viable and low-expertise route to the preparation of various geometry-tunable nano-apertures even though the mother Si master should be prepared by using the conventional semiconductor processes including the electron-beam lithography and focused ion-beam milling. Note that several hundreds of polymeric layers having multiscale apertures could be obtained from a single Si master. Depending on the use of a flat or a nano-patterned mould, a membrane with the two-level or three-level apertures was neatly formed with flexible, self-wetting characteristics, which enabled shadow masking in a step-and-repeat format with alignment. For the asymmetric nano-apertures, a simple design rule was derived. As a potential application, a facile method was also demonstrated with polymeric membranes by embedding the layer onto the tip of a syringe, yielding a highly uniform reorganization of water emulsions under a controllable manner. Materials Four commercially available UV-curable polymers (PUA301, PUA311, PFPE and NOA73) were used in the experiment. The hydrophilic PUA resin was composed of a functionalized prepolymer with acrylate groups for crosslinking a monomer, a photoinitiator and a radiation-curable releasing agent for surface activity. This material was purchased from Minuta Tech (Korea, MINS 301/311RM). The hydrophobic PFPE resin was purchased from Solvay Solexis (Italy, MD-700) and cured with a 3-wt% photoinitiator (Darocure 1173). The hydrophilic NOA73 was purchased from Norland Products Inc. (USA). Fabrication of a membrane with multilevel apertures A small amount of hydrophilic resin (PUA301, PUA311 and NOA73) was drop-dispensed onto a two-level hierarchical PFPE mould, and a flat or nano-patterned PFPE upper mould was uniformly placed onto the hierarchical mould. Then, the sandwich assembly was exposed to UV light (<3 min, λ =250~400 nm) under an applied pressure (25 g cm −2 ~1 kg cm −2 ) after forming conformal contact. After removal of the upper and lower PFPE moulds, a flexible, free-standing membrane with two-level or three-level apertures was obtained. To prepare a hydrophobic PFPE membrane, the same process was carried out by using the upper and lower moulds of PUA materials. Mechanical mapping of a binary surface made of two polymers The FMM measurement was performed with an AFM (XE-100, Park Systems, Korea) at the National Nanofab Center. The FMM mode with a constant set point of 1–5 nN was used at a scan rate of 1 Hz. The measured area was ~1.5 × 1.5 μm 2 . Facile emulsion reorganizations via individual apertures The pre-emulsion sample was prepared by mixing distilled water and hexadecane with 5% of surfactants (1:1 ratio of Span-20 and Tween-80, purchased from the Sigma-Aldrich). After gentle shaking, the solution having pre-emulsions was introduced via individual apertures by using a commercial syringe (1 ml min −1 ) to generate highly uniform nano-emulsions. How to cite this article: Cho, H. et al. Replication of flexible polymer membranes with geometry-controllable nano-apertures via a hierarchical mould-based dewetting. Nat. Commun. 5:3137 doi: 10.1038/ncomms4137 (2014).